A liquid crystalline chirality balance for vapours Chiral discrimination of vapours plays an important role in olfactory perception of biological systems and its realization by artificial sensors has been an intriguing challenge. Here, we report a simple method that tangibly visualizes the chirality of a diverse variety of molecules dissolved from vapours with high sensitivity, by making use of a structural change in a periodic microstructure of a nematic liquid crystal confined in open microchannels. This microstructure is accompanied by a topological line defect of a zigzag form with equal lengths of ‘zig’ and ‘zag.’ We find that a tiny amount of vapour of chiral molecules injected onto the liquid crystal induces the imbalance of ‘zig’ and ‘zag’ depending on its enantiomeric excess within a few seconds. Our liquid-crystal-based ‘chirality balance’ offers a simple, quick and versatile chirality-sensing/-screening method for gas-phase analysis (for example, for odours, environmental chemicals or drugs). Chiral discrimination of vapours plays an important role in olfactory perception of biological systems [1] , [2] . It has been an intriguing challenge to mimic such systems for the realization of artificial analogues such as odour sensors [3] , [4] for specific drug analysis and environmental monitoring. Many of the artificial gas sensors for chiral discrimination so far crucially rely on selective interactions between an analyte enantiomer and a complementary chiral environment. Construction of the latter, however, requires complex and ad-hoc molecular designs and syntheses, and therefore only molecules of specific architecture can be distinguished by these sensors. A nematic liquid crystal (NLC) is a fluid phase formed by anisotropic molecules that are preferentially aligned along a common axis n called the director [5] . It is well known that the sensitivity of the optical properties of NLCs to external stimuli has been effectively and ingeniously made use of in liquid crystal (LC) displays (here, the ‘external stimulus’ is an applied electric field), and NLCs have been an attractive candidate for chemical sensing as well. It is because they can exhibit optically-detectable changes in their macroscopic alignment when, for example, doped with chiral molecules [6] , [7] , [8] , [9] , [10] , [11] or analytes modify the surfaces of NLCs [12] , [13] . However, chiral sensing, especially of vapours, using NLCs has been a challenge because volatile small chiral molecules dissolved from a vapour phase can generally induce only a small change in the NLC alignment, which is difficult to detect. Although it was demonstrated half a century ago by Fergason [14] that the utility of a chiral NLC for sensing vapour molecules because the pitch of its helical alignment and the resulting structural colour are highly sensitive to the dissolution of vapour molecules, this mechanism cannot be used for chirality sensing, because the helical pitch varies irrespective of whether the absorbed molecules are chiral or not. Another reason why direct detection of the chirality of vapour samples using LC technology has not been achieved yet is that NLCs used for chirality detection are in most cases bounded by solid (or liquid) interfaces, which makes efficient dissolution of chiral molecules from their vapour phases practically impossible (a typical example is a Grandjean–Cano wedge cell [6] ). Still, self-organized non-trivial structures of a NLC confined in specific geometry [15] , [16] , [17] , [18] , [19] , [20] , [21] , [22] , [23] , [24] , [25] , [26] , [27] , [28] could enhance its response to a weak external stimulus so that the response could be manifest as the structural change directly observable using an optical microscope. Indeed, it has been reported that the curvature of a topological line defect in a twisted NLC cell is highly sensitive to chiral molecules doped in advance [10] . Here, as a possible means to detect the chirality of vapour samples, we consider an achiral NLC confined within an open microgroove [29] with frustrated interfacial alignment (anchoring) conditions. A great advantage of our open geometry is that vapour molecules readily dissolve into the NLC through the NLC/air interface, which is appropriate for efficient chirality detection. The NLC exhibits a topological line defect of the orientational order (a line disclination) of zigzag form [26] , [27] , [28] in the bulk ( Fig. 1a ). The formation of a line disclination is a manifestation of the frustrated anchoring conditions that do not allow a continuous orientation profile without singularities. The winding number [5] of the line disclination is +1/2, compatible with the anchoring conditions, and the curvature of the groove surface [28] . This zigzag line disclination is accompanied by self-organized periodic domains with alternating twist distortions along the vertical direction. In our previous work [26] , we showed that the twist distortions responsible for the formation of the zigzag line disclination is attributable to the smallness of the elastic constant K 22 for twist distortions compared with other elastic constants. The boundaries between domains with different twist directions involve a kink of the line disclination, as depicted schematically in Fig. 1a . Note that singularities of the orientational order in the NLC exist only at the line disclination; the kinks of the line disclination are not accompanied by any sheet-like singularities [5] . The length of a domain with right-handed twist distortion, l R , and that of a domain with left-handed twist distortion, l L , are equal because the free energy densities of both domains are the same (here the lengths are measured along the microgroove direction). This symmetry is attributed to the symmetry of the twist elastic energy, f t , with respect to the sign of the wavenumber of the twist distortion q ; f t =½ K 22 ( q − q 0 ) 2 , with q 0 being zero for achiral NLCs [5] . 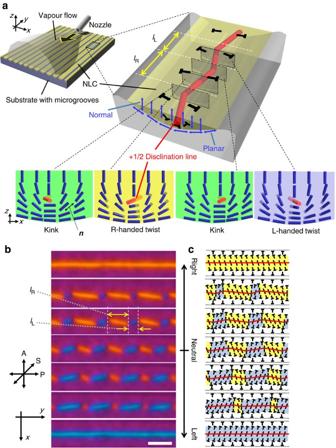Figure 1: Zigzag line defects and the chirality-specific responses to a chiral vapour. (a), Schematics of the experimental setup and zigzag line defects in a NLC confined within a microgroove of microwrinkles. Geometrical confinement and hybrid anchoring conditions (indicated by blue double-headed arrows) for a liquid filament of an NLC on a microwrinkle groove are shown. Blue cylinders illustrate the director structuresnaround different points of the zigzag line defect. The nail symbols (T) indicate the projection ofnonto the plane of the surface (the head of the nail comes out of the surface). The definition of the domain lengthslRandlLof the zigzag disclination line is shown. The analyte vapour is injected from a tube nozzle fixed to the substrate. The response is directly monitored by a POM. (b), Typical POM images for balanced and imbalanced zigzag domain lengths upon chiral vapour exposure (Scale bar, 10 μm). A sensitive tint plate is used with the configuration shown as S with the polarizer (P) and analyser (A). When the dissolved chiral molecules have the ability to induce right-/left-handed twist distortions, the length of domains with orange/blue colour increases and the imbalance is readily detected visually. (c), The director profiles below the line defect (The red line corresponds to the line defect, and the director profiles are shown by nail symbols. Yellow and blue regions are those with right-handed and left-handed twist distortions, respectively). Figure 1: Zigzag line defects and the chirality-specific responses to a chiral vapour. ( a ), Schematics of the experimental setup and zigzag line defects in a NLC confined within a microgroove of microwrinkles. Geometrical confinement and hybrid anchoring conditions (indicated by blue double-headed arrows) for a liquid filament of an NLC on a microwrinkle groove are shown. Blue cylinders illustrate the director structures n around different points of the zigzag line defect. The nail symbols (T) indicate the projection of n onto the plane of the surface (the head of the nail comes out of the surface). The definition of the domain lengths l R and l L of the zigzag disclination line is shown. The analyte vapour is injected from a tube nozzle fixed to the substrate. The response is directly monitored by a POM. ( b ), Typical POM images for balanced and imbalanced zigzag domain lengths upon chiral vapour exposure (Scale bar, 10 μm). A sensitive tint plate is used with the configuration shown as S with the polarizer (P) and analyser (A). When the dissolved chiral molecules have the ability to induce right-/left-handed twist distortions, the length of domains with orange/blue colour increases and the imbalance is readily detected visually. ( c ), The director profiles below the line defect (The red line corresponds to the line defect, and the director profiles are shown by nail symbols. Yellow and blue regions are those with right-handed and left-handed twist distortions, respectively). Full size image In general, the dissolution of chiral molecules into a NLC has the effect of transferring the molecular chirality to the macroscopic twisted/helical distortions of the director [5] , [6] , [7] , [8] , [9] , [10] , [11] . The presence of spontaneous twist distortions amounts to nonzero q 0 in f t . Let c ± denote the concentrations of (±)-enantiomers of a chiral molecule (the index indicates the sign of the predefined optical rotation), and q 0 is then written as q 0 = β + c + + β − c − = β ( c + − c − ). Here, chiral symmetry dictates that β + =− β − ≡ β . β is the twisting power, and its sign is defined such that β >0 when a (+)-enantiomer induces right-handed twist. Nonzero q 0 breaks the symmetry of f t with respect to q , and it is expected that, in our system with zigzag disclination lines, this asymmetry will manifest itself as unequal l R and l L , whose detection requires only a conventional polarized optical microscope (POM). Our experiments presented below clearly demonstrate that the dissolution of chiral molecules indeed brings about the structural change of a zigzag disclination line mentioned above, which is accounted for in a more quantitative manner by a simple theoretical model. The response is rapid enough because of the vapour dissolution/vaporization kinetics discussed below. The rapidness as well as high sensitivity of the response together with the simplicity of the setup makes our system useful as a simple method that tangibly visualizes the chirality of a diverse variety of vapour molecules. Responses of zigzag defects to a chiral vapour The setup of our experiments to substantiate the symmetry breaking of a zigzag disclination by chirality is sketched in Fig. 1 . The width w and the maximum thickness d of the NLC in the microgrooves are 12±1 μm and 1.8±0.2 μm, respectively. An analyte vapour is injected from a tube nozzle fixed near the surface of the NLC at a constant flow rate r , and the NLC surface is exposed to the steady flow for ~4 s for dissolution (see Methods). Without injection, the system is in contact with ambient air of relative humidity of ~50% at room temperature. The relative vapour concentration is c r = c v / c 0 , where c 0 is the concentration at the equilibrium vapour pressure at room temperature. The vapour injection tests were repeated with an interval of at least 10 min with an air flow for vaporization of the dissolved molecules. The sensor response is constantly monitored by the POM image with crossed polarizers. A sensitive tint plate is also used so that domains with left-handed twist are coloured in blue. Examples of microscope images with balanced and imbalanced zigzag domains, together with schematic illustrations of the orientational order, are shown in Fig. 1b,c . To characterize the resulting imbalance in the zigzag domain lengths, we introduce the enatiomeric excess of zigzag domains, that is, eez ≡ ( l R − l L )/( l R + l L ). In Fig. 2 , we show time-dependent raw responses of eez for saturated vapour mixtures ( c r =1) of (±)-limonene with different enantiomeric excesses of vapour, ee, defined by ee ≡ ( c + − c − )/( c + + c − ). In most cases, |eez| initially exhibits a rapid increase with time t and almost saturated in 4 s of exposure. After the cessation of vapour injection, |eez| decays rapidly with a characteristic time similar to that of the dissolution process, indicating the vaporization of dissolved molecules. 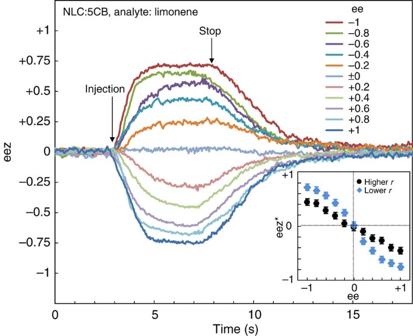Figure 2: Sensor signals upon exposure to limonene vapours. Time-dependent signals of imbalanced zigzag domain length, eez=(lR−lL)/(lR+lL), are shown for saturated limonene vapours with different enantiomeric excess, ee=(c+−c−)/(c++c−). Upon exposure to a stationary flow of chiral vapours with the flow rater=0.066 ml s−1, the signal magnitudes increase rapidly with time due to the dissolution, depending on ee, and are almost saturated in 4 s (seeSupplementary Discussion). After the injection is ceased, the signal magnitudes decay also quasi-exponentially towards the initial value due to evaporation. (Inset) The values of eez after 4 s exposure, denoted by eez*, are plotted against ee. The data for different flow ratesr=0.033 and 0.066 ml s−1are shown. As a NLC, pentylcyanobiphenyl (5CB) is used here. Figure 2: Sensor signals upon exposure to limonene vapours. Time-dependent signals of imbalanced zigzag domain length, eez=( l R − l L )/( l R + l L ), are shown for saturated limonene vapours with different enantiomeric excess, ee=( c + − c − )/( c + + c − ). Upon exposure to a stationary flow of chiral vapours with the flow rate r =0.066 ml s −1 , the signal magnitudes increase rapidly with time due to the dissolution, depending on ee, and are almost saturated in 4 s (see Supplementary Discussion ). After the injection is ceased, the signal magnitudes decay also quasi-exponentially towards the initial value due to evaporation. (Inset) The values of eez after 4 s exposure, denoted by eez*, are plotted against ee. The data for different flow rates r =0.033 and 0.066 ml s −1 are shown. As a NLC, pentylcyanobiphenyl (5CB) is used here. Full size image Now let us estimate the characteristic time τ of relaxation of the director orientation that is given by τ ~ η 0 d 2 / K (for example, ref. 5 ), with d , η 0 and K being the characteristic length, the effective viscosity and the typical elastic constant, respectively. With d ~1 μm (thickness of the NLC filament), η 0 ~10 −3 Pa s and K ~10 −11 N, τ is estimated as ~10 −3 s. This is much shorter than the timescale of the observed response, a few seconds; the director reorientation well follows the concentration change of the chiral dopant within the experimental timescale of interest. Even when the length of ‘zig’ or ‘zag’ part (10 μm at most from Fig. 1 ) is taken as d , the estimated τ ~ 10 −1 s is still smaller than a few seconds. Therefore, the relaxation of the orientational order (and hence the defects) plays essentially no role in the determination of the characteristic response time and the observed response directly reflects the concentration change governed by the dissolution/evaporation kinetics through the air-NLC interface ( Supplementary Discussion ). The observed response shown in Fig. 2 also suggests that the vapour dissolution/vaporization kinetics is a first-order process ( Supplementary Discussion ). As, in our very thin NLC, the characteristic time should be proportional to d , the quick response of a few seconds owes to the present small spatial scale of the LC confined within microgrooves. A change in |eez| of ~0.2 in such a timescale is readily detected by observing which twisted domains elongate or shrink ( Supplementary Movie 1 ). Additional experiments ( Supplementary Fig. 1 ) indicate that our method enables the detection of induced helical pitch ( ∝ q 0 ) as large as 0.1~1 mm, demonstrating high sensitivity to a chirality-induced structural change. Responses to various chiral vapours The sign of β is material dependent, and the present results indicate β <0 for (+)-limonene-rich analytes because they elongate left-handed twist domains. This information is important for the identification of the chirality of analytes, that is, the absolute stereochemical configuration, and is most easily obtained by the present method. Table 1 shows the results for various chiral vapours including major aroma constituents, demonstrating the versatility of the present method. As references, we have also confirmed that achiral vapours, for example, p -menthane and vanillin, yield no detectable change in eez. Table 1 Sign of β determined by the present liquid crystal (LC)-based chirality sensor. Full size table The amount of analyte vapours necessary for chiral detection is significantly small owing to the quick response; only a volume of ~0.26 ml was injected within 4 s for each curve shown in Fig. 2 . In addition, the quick vaporization also reduces the waiting time for the next test, which is accelerated further by exposure of the NLC to air flow. The values of eez after 4 s exposure are plotted against ee in inset in Fig. 2 . Again this confirms that β <0 for (+)-limonene because d (eez)/ d (ee)<0. Point symmetry of the plots with respect to the origin indicates that the present system directly detects the imbalance and the sign of the chirality, and only the knowledge of the sign of β ( Table 1 ) is required as perquisite to discriminate enantiomers. This mechanism is entirely different from that of other conventional chiral sensing [3] , [4] and analytical methods, such as chiral chromatography techniques [30] , which require the complementary chiral environments for respective enantiomers. The effect of the flow rate r on the responses of eez is also clearly shown; the sensitivity of eez to ee increases with r owing to the enhanced dissolution. By exploiting the plots in inset in Fig. 2 as calibration curves, we can quantify ee of a vapour sample containing (±)-enantiomers of a single species from the observed response at fixed time t , c v and r . Additional experiments ( Fig. 3 ) demonstrate the ability to quantify c r for different enantiopure chiral compounds, that is, |ee|≈1. The plots of |eez| at t =4 s and r =0.33 ml s −1 with respect to c r also show sublinear dependence with respect to c r and the saturation of |eez|→1 at higher concentrations. These plots can be exploited as calibration curves for the determination of the vapour concentration of the pure enantiomer. The chiral material-dependent curves indicate the difference in the sensitivity; β pinene>limonene>carvone>terpinen-4-ol>menthol. The sensitivity depends on various material-dependent unknown parameters, such as those for dissolution/vaporization kinetics and β , and is difficult to estimate in advance. Nevertheless, once the curves are acquired, the difference would be a useful clue to estimate the major compound especially for a mixture of chiral compounds. Accordingly, the detection limit is also material dependent; for example, the minimum detectable value of c r for carvone is approximately 0.01 corresponding to ~5 p.p.m. This is comparable to or better than that of the previously reported method based on a field effect transistor [4] . 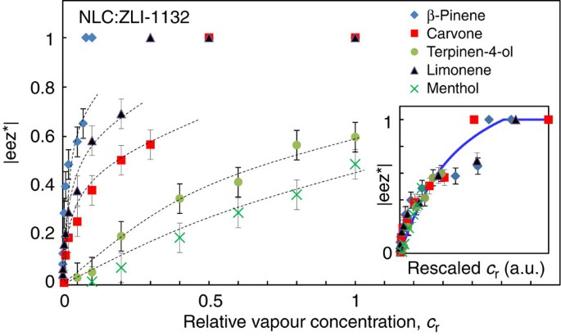Figure 3: Vapour-concentration-dependent signals of LC-based chirality. The values of eez* (mean±r.m.s.) are plotted against relative vapour concentrationcrfor different chiral vapours of enatiopureβ-pinene, limonene, carvone, terpinen-4-ol and menthol. The flow rateris 0.33 ml s−1. As a NLC, ZLI-1132 is used here. Broken lines are guides for visibility. Forβ-pinene, limonene and carvone, the eez* values are saturated at highercr. The detection limits for, for example,β-pinene and carvone are very low;cr~0.001 and 0.01, corresponding to ~3 and ~5 p.p.m., respectively. Using the plots here as the calibration curves, ee orcrcan be estimated for the analyte vapours for fixed flow rate. (Inset) The identical data are plotted with rescaledcr, demonstrating the universality of the response curves with sublinear dependence of eez on the chiral vapour concentration. The theoretically predicted curve (see Methods) is also shown as a solid blue line, indicating the qualitative agreement. Figure 3: Vapour-concentration-dependent signals of LC-based chirality. The values of eez* (mean±r.m.s.) are plotted against relative vapour concentration c r for different chiral vapours of enatiopure β -pinene, limonene, carvone, terpinen-4-ol and menthol. The flow rate r is 0.33 ml s −1 . As a NLC, ZLI-1132 is used here. Broken lines are guides for visibility. For β -pinene, limonene and carvone, the eez* values are saturated at higher c r . The detection limits for, for example, β -pinene and carvone are very low; c r ~0.001 and 0.01, corresponding to ~3 and ~5 p.p.m., respectively. Using the plots here as the calibration curves, ee or c r can be estimated for the analyte vapours for fixed flow rate. (Inset) The identical data are plotted with rescaled c r , demonstrating the universality of the response curves with sublinear dependence of eez on the chiral vapour concentration. The theoretically predicted curve (see Methods) is also shown as a solid blue line, indicating the qualitative agreement. Full size image As examples of a simple analysis of natural vapour mixtures, we determined the signs of eez for the headspace gases taken from vials containing torn orange ( Citrus unshiu ) peels, torn spearmint ( Mentha spicata ) leaves and torn immature conifer cone of a Japanese red pine ( Pinus densiflora ) to be (−), (+) and (+), respectively. If we assume that the major volatile compounds for the orange peel is limonene, that for the spearmint is carvone and those for the pine conifer cone are α / β -pinenes [31] , the signs of their optical rotations are reasonably estimated from the obtained signs of β for (+)-enantiomers ( Table 1 ); (+)-limonene, (−)-carvone and (−)- α / β -pinenes. Finally, we discuss the behaviour of l R and l L in response to nonzero q 0 . We begin with our previous model accounting for the occurrence of a zigzag disclination in an achiral NLC [26] , and extend it to include the effect of chirality. Refer to Methods for details of the theoretical argument. We find that |eez| increases sublinearly with the increase of | q 0 | until it reaches 1, in qualitative agreement with our experimental results ( Fig. 3 ). Moreover, the experimental curves fall well onto a single theoretical curve after appropriate rescaling of c (Inset of Fig. 3 ). Though admittedly crude, our theoretical model accounts for our experimental findings remarkably well. The presence of a master curve shown in the inset of Fig. 3 clearly demonstrates the universality of the chirality-induced symmetry breaking of the zigzag defect, which could be used as a standard for a diverse variety of chiral vapours such as essential oils, aroma constituents and phytoncides. To conclude, we have shown for the first time that it is possible to detect the existence of chirality in vapour samples with high sensitivity, by making use of a structural change in a periodic microstructure of an achiral NLC confined in open microchannels. Although it is already known that the pitch of a cholesteric LC, and thus its colour, change according to the sign of the chirality of dissolved chiral molecules [5] , the variation of the pitch cannot be applied to the determination of the existence of chirality because the pitch can vary sensitively in response to the dissolution of achiral [14] as well as chiral molecules. Therefore, we stress the advantage of our method over the previous ones based on LCs in that the distinction between chiral and achiral molecules is possible. In addition, our system works at ambient temperature and pressure, and its setup is highly simple and not at all demanding; sinusoidal microgrooves, an achiral NLC of volume less than 1 pl, and an ordinary POM. Moreover, it requires only a few ml of collected or prepared gas-phase analyte for chiral sensing and no condensation, extraction or predissolution into a solvent is necessary. Our zigzag disclination line that responds to the presence of chirality with clear structural changes could be dubbed ‘a chirality balance,’ and offers a simple, quick and economical chirality-sensing method, especially suitable for vapour samples, facilitating the construction of a portable and user-friendly chiral sensor. In addition, our method as an optional chiral-screening technique could complement conventional gas-phase analyses such as gas chromatography [30] . Preparation of zigzag defects in a NLC Microwrinkles with aligned microgrooves filled with a NLC that shows a zigzag defect structure were prepared according to the identical protocols reported in ref. 26 . The microwrinkles were self-organized on the top surface of a polyimide-capped polydimethylsiloxane substrate (12 × 12 × 6 mm 3 ). The wavelength of the groove λ was 14.5 μm. The aspect ratio of the microwrinkles was almost constant, 0.13±0.01. The microgrooves were filled with room temperature NLCs, by spreading a droplet of the NLC placed on the microgrooved surface. With the present aspect ratio, pentylcyanobiphenyl (Sigma-Aldrich) or ZLI-1132 (MERCK) was stabilized within the microgrooves via capillary effect [29] . The air/liquid and wrinkle/liquid interfaces impose normal anchoring and unidirectional planar anchoring, respectively. The local easy axis of the latter is perpendicular to the groove direction and along tangential direction of the sinusoidal curve on the plane. These antagonistic anchoring conditions lead to frustrated alignment with a wedge disclination line of topological charge +1/2, which spontaneously shows zigzags. The LC alignment was observed using a transmitted polarized microscope (BX-51P, Olympus). To differentiate small optical rotations visually by the colour difference, a 530 nm sensitive tint plate (1λ, U-TP530, Olympus) was used as a test plate compensator under crossed-Nicol conditions. Preparation of analyte vapours We prepared a vial (40 ml) with a rubber septum containing 1–5 g of a volatile liquid or solid compound with chirality. The headspace was equilibrated at least for 15 min with rotating magnetic stirrer before sampling. For limonene, 11 mixtures with ee from −1 to +1 with the intervals of 0.2 were prepared by mixing the enantiopure enantiomers, (±)-limonene (Sigma-Aldrich). To prepare diluted vapours, the saturated one was mixed with air with vigorous stirring. Enantiopure compounds used in this study are 2,3-butanediol, 1-phenylethanol, α -pinene, 3-carene, carvone, carveol, menthone, limonene, borneol, linalool, β -citronellol, trans -caryophyllene, 2-butanol, camphene, α -thujone, fenchone, rose oxide, menthol, menthyl chrolide, menthyl acetate and α -bisabolol (Sigma-Aldrich), and terpinen-4-ol (TCI), and 1-phenylethylamine, β -pinene, δ -decanolactone, α -terpineol and ibuprofen (WAKO chemical). Achiral compounds, p -menthane and vanillin (Sigma-Aldrich) were also used as analyte vapour compounds to confirm that the present LC-based chirality sensor show no response to them. Three natural plant-based chiral vapour mixture samples were prepared as follows. The peels of a fresh orange ( Citrus unshiu ), fresh spearmint ( Mentha spicata ) leaves and fresh yellow-greenish immature conifer cone of a Japanese red pine ( Pinus densiflora ) were torn and approximately 2 g of each was put into an individual vial with rubber septa. The vapour mixtures were sampled for tests from the headspace after a 10-min equilibration. Experimental setup The nozzle of a Teflon tube with an inner diameter of 0.5 mm was fixed above the LC surface. The flow axis was inclined and made an angle of 14° with the surface. The flow rate r was controlled by the injector between 0.033 and 0.33 ml s −1 . Soon after 4 ml of an analyte vapour was sampled into a disposable syringe (5 ml, SS-05LZ, Termo) from the headspace of the sample vial, the syringe was connected to the Teflon tube through the syringe needle. The injection, which was electrically controlled using a stepping motor (SGSP-25ACT-B0, Sigma-Koki), was initiated within 1 min after vapour sampling and it was kept for 4 s. After the cessation of injection, the dissolved molecules could evaporate because the NLC was now exposed to an ambient atmosphere. POM images were monitored and zigzag domains lengths were measured by tracking the domain boundaries from the acquired movies (30 frames/s) by a software analysis (2D-PTV, Digimo). Five pairs of analysed zigzag domain lengths were averaged to calculate eez. The observed position was fixed to an area, which was approximately 1.5 mm apart from the nozzle along the nozzle axis. The NLC with the zigzag defects could be repeatedly used for the sensing by expelling the dissolved volatile molecules after each test by air flow or heat and was stable for at least 6 months in an ambient condition. Theoretical model To discuss the free energy of the NLC with a zigzag defect, we consider three contributions; (i) the elastic energy of a (straight) disclination line E ( Ω ), as a function of its angle with respect to the groove direction ( Ω ), (ii) the energetic penalty of the disclination line approaching the groove wall f 1 , and (iii) the free energy of defect kinks f 2 (in the following, ε , f 1 and f 2 are the free energies per unit length of the groove). To evaluate E ( Ω ), we start with the elastic energy of a disclination line given in equation (1) of ref. 26 for an achiral NLC, that is, and discuss how Equation (1) is extended to the case of a chiral nematic. Here, φ characterizes the twist distortions below the disclination line, γ is the anchoring strength at the groove surface, κ ≡ (π K /4)ln( R / r c ). K is the splay/bend elastic constant (they are assumed to be equal for simplicity), and R and r c are the upper/lower cutoff, respectively, for the evaluation of the elastic energy of the disclination line (See ref. 26 . R is determined by the depth of the LC, and r c is the size of the disclination core). The first term, the contribution from the elastic distortions around the disclination line (with microscopic cutoff r c and the outer cutoff R ) is not affected by chirality. The second term taking care of the contribution from twist distortions is now modified to (1/2) γ ( φ − q 0 ) 2 , where q 0 is the wavenumber of spontaneous twist distortions arising from chirality (defined in the main text), and is the thickness of the region in which twist distortions are relevant (see Fig. 4a of ref. 26 , where is denoted by d ). 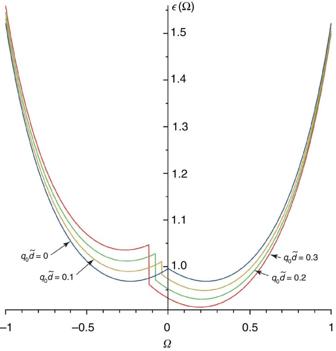Figure 4: Elastic energy of a disclination line. Here, we plot the elastic energy of a disclination lineεas a function of its angleΩwith respect to the groove direction for different strengths of chirality denoted byq0. See Methods for the evaluation ofε. Figure 4: Elastic energy of a disclination line. Here, we plot the elastic energy of a disclination line ε as a function of its angle Ω with respect to the groove direction for different strengths of chirality denoted by q 0 . See Methods for the evaluation of ε . Full size image We minimize ε ( Ω , φ ) with respect to φ numerically, and plot ε ( Ω ) for various values of q 0 in Fig. 4 . We observe (i) that ε ( Ω )→∞ when Ω →π/2 (which is obvious from Eq. (1)), (ii) that the value of Ω giving the minimum of ε ( Ω ), which will be denoted by Ω 0 hereafter, is insensitive to the variation of q 0 , (iii) convex form of ε ( Ω ) around Ω 0 , and (iv) ε ( Ω 0 )≈− ε (− Ω 0 ). From these observations, we can safely model ε ( Ω ) by, which facilitates the following numerical analyses. Here, η is a numerical constant of order unity, and Δ characterizes the strength of chirality. ( Δ =0 for an achiral case). With a reasonable choice of α c =0.1, K 22 / K =0.5, γ / κ =0.2, we have η ≈1, Ω 0 ≈0.2. We also note that Δ is almost proportional to q 0 , and Δ / q 0 ≈−0.17 for the above choice of parameters. f 1 has been already presented in ref. 26 and in the present notation, it reads where g 1 ( x ) ≡ x −1 ln[(1+ x )/(1− x )], λ is the width of the groove, and D ≡ ( l /2) × tan Ω , with l being the length of the projection of a segment of line disclination onto the groove direction. When c 1 ≈1 and K ≈ κ , c 1 Kh /( λ /2)= α κ with α ≈0.25. In the following, we measure the length in units of λ /2. As we did in ref. 26 , we simply assume that the elastic energy per kink is f 2 ≈ κ l d , where l d has the dimension of length and is assumed to be small compared with other relevant characteristic lengths. The energetics of a disclination line with ‘asymmetric’ zigzag form is now given as follows. The ‘zig’ part is characterized by l = l R and D = D R (and tan Ω R =2 D R / l R ), and the ‘zag’ part by l = l L and D = D L . Then the total energy of a zigzag disclination line per unit length of the groove is given by Note again that all the lengths are measured in units of λ/2 and D R,L , l R,L and l d are now dimensionless. We minimize f zigzag with respect to D R,L and l R,L . Note that D R + D L must be zero because otherwise the zigzag disclination will eventually reach the wall of the groove. From our experimental observations, we find that the number of kinks per unit length stays constant except when a first-order transition occurs between a disclination with kinks and a straight one. The constancy of the number of kinks is probably attributed to a large energy barrier for the creation or annihilation of kinks. Therefore, we impose l R + l L =(const.) in addition when we minimize f zigzag . We determine the constant l R + l L by minimizing f zigzag for Δ =0 with the constraint D R + D L =0 and no constraint for l R,L (in this case l R = l L ). In the inset of Fig. 3 , we plot eez ≡ ( l R – l L )/( l R + l L ) as a function of Δ for α =0.25, η =1, Ω 0 =0.2 and l d =0.04. Δ is appropriately rescaled to compare this theoretical eez to experimental ones. This theoretical argument nicely reproduces some qualitative features of the experimental eez; sublinear dependence of eez on c r ( ∝ q 0 ) and the saturation of eez to 1 for large c r . How to cite this article: Ohzono, T. et al. A liquid crystalline chirality balance for vapours. Nat. Commun. 5:3735 doi: 10.1038/ncomms4735 (2014).